Modulation of dopamine release in the striatum by physiologically relevant levels of nicotine Striatal dopamine (DA) release can be independently triggered not only by action potentials (APs) in dopaminergic axons but also APs in cholinergic interneurons (ChIs). Nicotine causes addiction by modulating DA release, but with paradoxical findings. Here, we investigate how physiologically relevant levels of nicotine modulate striatal DA release. The optogenetic stimulation of ChIs elicits DA release, which is potently inhibited by nicotine with an IC 50 of 28 nM in the dorsal striatum slice. This ChI-driven DA release is predominantly mediated by α6β2* nAChRs. Local electrical stimulus (Estim) activates both dopaminergic axons and ChIs. Nicotine does not affect the AP DA -dependent DA release (AP DA , AP of dopaminergic axon). During burst Estim, nicotine permits the facilitation of DA release by prevention of DA depletion. Our work indicates that cholinergic stimulation-induced DA release is profoundly modulated by physiologically relevant levels of nicotine and resolves the paradoxical observation of nicotine’s effects on striatal DA release. Nicotine is the psychoactive component causing tobacco addiction. After cigarette smoking, nicotine increases up to 300 nM in the plasma and rapidly permeates into the brain [1] . The dopamine (DA) system, which is responsible for many behaviours such as reward signalling, reinforcement and locomotor activity, is profoundly involved in nicotine addiction. Nicotine not only excites midbrain dopaminergic neurons by activating nicotinic acetylcholine receptors (nAChRs) on the dopaminergic somata and by modulating synaptic inputs [2] , [3] , [4] , [5] , but also modulates terminal DA release in the forebrain. By using electrical-field stimulation (Estim), nicotine was found to suppress the striatal DA release evoked by single action potentials (APs) and to enhance the contrast between DA release evoked by phasic and tonic firing [6] , [7] , [8] . These observations are explained by the desensitization of nAChRs on the dopaminergic terminals and the reduction of short-term depression. The striatum, comprising the dorsal striatum and the nucleus accumbens (NAc, ventral striatum), is the major region in the forebrain for terminal DA release [9] , [10] , which can be recorded in real time by either electrochemical voltammetry or amperometry with a carbon fibre electrode (CFE) [11] , [12] , [13] . It was discovered long ago that DA in the striatum is released from widespread axonal arbours whose somata are located in the distant midbrain (the ascending pathway). Recent studies discovered that, independent of the AP firing of dopaminergic somata/axons, the AP firing of striatal cholinergic interneurons (ChIs) also drives DA release [14] , [15] , [16] . This local axon-axon pathway is termed as the ‘ChI pathway’. Currently, it is a common view that DA release from the ascending pathway is modulated by nicotine [6] , [7] , [8] , [17] . However, this conclusion was made from studies based on Estim without considering a possible contribution of the ChI-driven DA release. Since the AP of ChIs is as important as the AP of dopaminergic axons in triggering DA release, whether the ChI pathway contributes to the known nicotinic modulation of DA release is an essential open question. nAChRs on dopaminergic terminals belong to two classes: α6β2* and α4(non-α6)β2* (*denotes the possible presence of other subunit) [18] , [19] , [20] , [21] , [22] . Previous studies suggested that β2* nAChRs mediate ChI-driven DA release [14] , [15] . α6* nAChRs are known to modulate DA release [18] , [22] , [23] , [24] , but whether/how α6* nAChRs trigger DA release remains unknown. In the present work, we revisited the mechanisms underlying nicotine’s effect on DA release in dorsal striatum slices. We separated the signal of DA release via the two pathways in ChAT-ChR2-EYFP transgenic mice, which selectively express the light-gated cation channel channelrhodopsin-2 (ChR2) in the cholinergic neurons. Surprising, the ChI-driven DA release was highly sensitive to acute exposure to physiologically relevant levels of nicotine, while the DA release driven by AP firing of dopaminergic axons was insensitive to nicotine. By suppressing the ChI pathway and reducing the ChI-induced depletion of DA vesicle pool, physiologically relevant levels of nicotine facilitated the later DA release during sustained burst Estim in striatum, which could be a mechanism underlining reward seeking in smokers. Nicotine inhibits ChI-driven DA release In dorsal striatum slices from ChAT-ChR2-EYFP transgenic mice, ChR2-EYFP was strongly expressed on the cell membrane of all neurons, which were labelled by antibody against vesicular acetylcholine transporter (VAChT, a marker of ChIs; Fig. 1a ). When transient light stimulation (Lstim, 1 ms in duration) was applied to the slice, AP firing was recorded under current-clamp in the ChIs that were identified by EYFP fluorescence ( Fig. 1b upper). However, Lstim did not affect the membrane potential of midbrain dopaminergic neurons that were ChR2-EYFP negative (data not shown). These results suggested that optogenetic stimulation precisely and selectively evoked AP firing activity of striatal ChIs in ChAT-ChR2-EYFP transgenic mice. We recorded DA release in the striatum by electrochemical amperometry with CFEs. When a transient Lstim was applied to the striatal slice, there was an increase in amperometric current I amp (Lstim), representing the signal of extracellular DA increase ( Fig. 1b lower). As ChI-driven DA release, I amp (Lstim) was induced by the AP firing of the cholinergic somata/axons (through the ChI pathway) [14] , [15] , [16] . 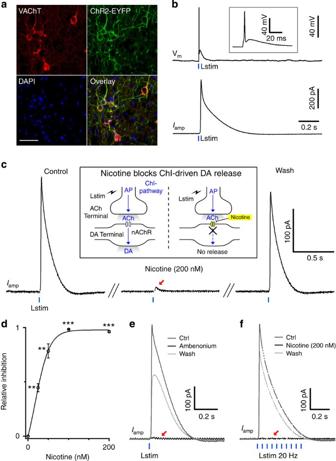Figure 1: Physiologically relevant levels of nicotine inhibit DA release triggered by cholinergic interneurons (ChIs) in the dorsal striatum. (a) Specific expression of ChR2-EYFP in striatal ChIs identified by the expression of vesicular ACh transporter (VAChT). Scale bar, 50 μm. (b) A transient light stimulus (Lstim, 1 ms in duration) evoked an AP in a current-clamped ChI (−200 pA current was injected to silence basal firing,n=11; upper) and Lstim-induced DA release (Iamp(Lstim), n=40; lower). Inset: the AP on an expanded scale. (c) DA release induced by a single pulse of Lstim was reversibly inhibited by 200 nM nicotine (n=18). Inset: physiologically relevant levels of nicotine blocked ChI-driven DA release. (d) Dose–response relationship of the nicotine’s effect onIamp(Lstim). Data points are fitted by a sigmoid function with an IC50of 28 nM (n=4 for 25 and 50 nM, 3 for 100 nM, 18 for 200 nM). Note that the pretreatment time was 20–30 min for 25–100 nM and 5–10 min for 200 nM. (e) Ambenonium (100 nM), an antagonist of acetylcholinesterase, reversibly inhibited Lstim-induced DA release (n=4). (f) DA release induced by a train of Lstim at 20 Hz was reversibly inhibited by 200 nM nicotine (n=5). **P<0.01, ***P<0.001, pairedt-test. Data are mean±s.e.m. Figure 1: Physiologically relevant levels of nicotine inhibit DA release triggered by cholinergic interneurons (ChIs) in the dorsal striatum. ( a ) Specific expression of ChR2-EYFP in striatal ChIs identified by the expression of vesicular ACh transporter (VAChT). Scale bar, 50 μm. ( b ) A transient light stimulus (Lstim, 1 ms in duration) evoked an AP in a current-clamped ChI (−200 pA current was injected to silence basal firing, n =11; upper) and Lstim-induced DA release ( I amp (Lstim), n=40; lower). Inset: the AP on an expanded scale. ( c ) DA release induced by a single pulse of Lstim was reversibly inhibited by 200 nM nicotine ( n =18). Inset: physiologically relevant levels of nicotine blocked ChI-driven DA release. ( d ) Dose–response relationship of the nicotine’s effect on I amp (Lstim). Data points are fitted by a sigmoid function with an IC 50 of 28 nM ( n =4 for 25 and 50 nM, 3 for 100 nM, 18 for 200 nM). Note that the pretreatment time was 20–30 min for 25–100 nM and 5–10 min for 200 nM. ( e ) Ambenonium (100 nM), an antagonist of acetylcholinesterase, reversibly inhibited Lstim-induced DA release ( n =4). ( f ) DA release induced by a train of Lstim at 20 Hz was reversibly inhibited by 200 nM nicotine ( n =5). ** P <0.01, *** P <0.001, paired t -test. Data are mean±s.e.m. Full size image To determine the effect of nicotine on the ChI-driven DA release, we applied physiologically relevant levels of nicotine (25–200 nM) to the striatal slice. The Lstim-induced DA release was reversibly and potently inhibited by 96±1% after pretreatment with 200 nM nicotine for ≤10 min ( Fig. 1c ). The median inhibitory concentration (IC 50 ) was 28 nM ( Fig. 1d ). The nicotinic inhibition of I amp was most likely caused by the desensitization of nAChRs [6] , [7] , [8] . To confirm this, we challenged the striatal slice with 100 nM ambenonium, an inhibitor of acetylcholinesterase. In the presence of ambenonium, nAChRs on the dopaminergic terminals should be desensitized by the accumulated extracellular acetylcholine, leading to the blockade of ChI-driven DA release. Indeed, after pretreatment with ambenonium, Lstim-induced DA release was inhibited to 13±7% of control ( Fig. 1e ). In addition to the DA release induced by a single pulse of Lstim, the release induced by a train of Lstim at 20 Hz was also completely inhibited by 200 nM nicotine ( Fig. 1f ). These results suggested that the DA release induced by either tonic or phasic activity of the ChIs was inhibited by acute exposure to physiologically relevant levels of nicotine. α6β2* nAChRs mediate ChI-driven DA release To identify the subunits of nAChRs involved in ChI-driven DA release via the ChI pathway, we measured Lstim-induced DA release in the presence of a selective antagonist for either α6* or β2* nAChRs. We challenged the slice with α-conotoxin MII (α-ctx MII), a selective antagonist of α6* nAChRs [17] , [25] . The I amp (Lstim) was reversibly inhibited to 13±3% after pretreatment with 100 nM α-ctx MII and recovered to 42±4% after washout ( Fig. 2a,c left). We also confirmed that dihydro-β-erythroidine hydrobromide, a selective antagonist of β2* nAChRs [26] , potently inhibited I amp (Lstim) to 2.0±0.3%. The signal recovered to 80±10% after washout ( Fig. 2b,c right). These results suggested that the ChI-driven DA release was predominantly mediated by α6β2* nAChRs on dopaminergic terminals. 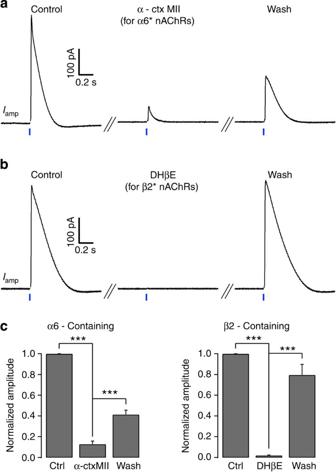Figure 2: α6β2* nAChRs are responsible for ChI-driven DA release. (a) The Lstim-induced DA release was inhibited by pretreatment with 100 nM α-conotoxin MII (α-ctx MII, a selective antagonist of α6* nAChRs, *denotes the possible presence of other subunits) for 15 min, and partial recovered after washout for 1–1.5 h. (b) The Lstim-induced DA release was inhibited by pretreatment with 1 μM dihydro-β-erythroidine hydrobromide (DHβE, a selective antagonist of β2* nAChRs) for 15 min, and recovered after washout for a prolonged period of 1–2 h. (c) Summary histograms of experiments shown in panelsaandb. Left, the Lstim-induced DA release was inhibited by 87±3% by α-ctx MII, and recovered to 42±4% of the control level after washout (n=8). Right, the Lstim-induced DA release was inhibited by 98±0.3% by 1 μM DHβE, and recovered to 80±10% of the control level after washout (n=6). ***P<0.001, pairedt-test. Data are mean±s.e.m. Figure 2: α6β2* nAChRs are responsible for ChI-driven DA release. ( a ) The Lstim-induced DA release was inhibited by pretreatment with 100 nM α-conotoxin MII (α-ctx MII, a selective antagonist of α6* nAChRs, *denotes the possible presence of other subunits) for 15 min, and partial recovered after washout for 1–1.5 h. ( b ) The Lstim-induced DA release was inhibited by pretreatment with 1 μM dihydro-β-erythroidine hydrobromide (DHβE, a selective antagonist of β2* nAChRs) for 15 min, and recovered after washout for a prolonged period of 1–2 h. ( c ) Summary histograms of experiments shown in panels a and b . Left, the Lstim-induced DA release was inhibited by 87±3% by α-ctx MII, and recovered to 42±4% of the control level after washout ( n =8). Right, the Lstim-induced DA release was inhibited by 98±0.3% by 1 μM DHβE, and recovered to 80±10% of the control level after washout ( n =6). *** P <0.001, paired t -test. Data are mean±s.e.m. Full size image Estim evokes DAergic AP-dependent and ChI-driven DA release In contrast to Lstim-induced DA release, the DA release induced by Estim had a remarkable inflection point in the onset of I amp (Estim). This inflection point divided the onset of I amp (Estim) into two phases: phase I before the point and the phase II after the point ( Fig. 3a ). These two phases probably occurred because local Estim simultaneously stimulated both the dopaminergic axons and the ChIs. The I amp (Lstim) and the phase II component of I amp (Estim) showed nearly the same temporal profile (indicated by the dashed lines) suggesting that, like I amp (Lstim), the phase II component of I amp (Estim) originated from the ChI pathway ( Fig. 3a ). This was further confirmed by the finding that both I amp (Lstim) and the phase II of I amp (Estim) were totally blocked by 10 μM mecamylamine (MEC), a non-selective antagonist of nAChR, while the phase I of I amp (Estim) remained intact in the presence of MEC ( Fig. 3b,d ). These results demonstrated that local Estim stimulated not only the dopaminergic axons but also the ChIs in the dorsal striatum slices. The AP of dopaminergic axons directly drove the phase I component of DA release of dopaminergic terminals, while the AP of ChIs indirectly drove the phase II component of I amp (Estim). 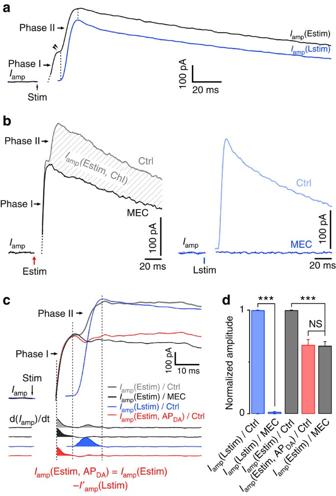Figure 3: Electrical-field stimulation (Estim)-induced mixed-DA release driven by APs of dopaminergic axons and ChIs. (a) Following Estim, but not Lstim, there was an ‘inflection point’ (double arrows) during the onset of the DA release signal. DA release (Iamp) before and after the inflection point was identified as the phase I and the phase II components. The identical latency betweenIamp(Lstim) and phase II ofIamp(Estim) (indicated by the dashed lines) implicated that the phase II component ofIamp(Estim) was probably from the same source asIamp(Lstim). (b) The DA release via the ChI pathway induced by either Estim (phase II ofIamp(Estim), left) or Lstim (Iamp(Lstim), right) was blocked by 10 μM mecamylamine (MEC, 30 min pretreatment), a non-selective antagonist of nAChRs44. However, phase I ofIamp(Estim) was intact in the presence of MEC, suggesting that the phase I signal reflected DA release driven by AP of dopaminergic axons (Iamp(Estim, APDA)), while the phase II signal reflected DA release driven by AP of ChIs (Iamp(Estim, ChI);n=11). All recordings from the same cell. (c) The phase I componentIamp(Estim, APDA) was isolated from totalIamp(Estim) asIamp(Estim, APDA)=Iamp(Estim)−Iamp(Estim, ChI).Iamp(Estim, ChI) was estimated byI'amp(Lstim), which wasIamp(Lstim) normalized to the phase II amplitude ofIamp(Estim). Note, the amplitude and phasic timing of the mathematically isolatedIamp(Estim, APDA) was equal to that of the totalIamp(Estim) in the presence of 10 μM MEC. (d) Summary of theIamp(Lstim) andIamp(Estim) with and without 10 μM MEC, as well asIamp(Estim, APDA). The data shown in panelsb–dwere from the same cells (n=11). ***P<0.001, pairedt-test. Data are mean±s.e.m. Figure 3: Electrical-field stimulation (Estim)-induced mixed-DA release driven by APs of dopaminergic axons and ChIs. ( a ) Following Estim, but not Lstim, there was an ‘inflection point’ (double arrows) during the onset of the DA release signal. DA release ( I amp ) before and after the inflection point was identified as the phase I and the phase II components. The identical latency between I amp (Lstim) and phase II of I amp (Estim) (indicated by the dashed lines) implicated that the phase II component of I amp (Estim) was probably from the same source as I amp (Lstim). ( b ) The DA release via the ChI pathway induced by either Estim (phase II of I amp (Estim), left) or Lstim ( I amp (Lstim), right) was blocked by 10 μM mecamylamine (MEC, 30 min pretreatment), a non-selective antagonist of nAChRs [44] . However, phase I of I amp (Estim) was intact in the presence of MEC, suggesting that the phase I signal reflected DA release driven by AP of dopaminergic axons ( I amp (Estim, AP DA )), while the phase II signal reflected DA release driven by AP of ChIs ( I amp (Estim, ChI); n =11). All recordings from the same cell. ( c ) The phase I component I amp (Estim, AP DA ) was isolated from total I amp (Estim) as I amp (Estim, AP DA )= I amp (Estim)− I amp (Estim, ChI). I amp (Estim, ChI) was estimated by I ' amp (Lstim), which was I amp (Lstim) normalized to the phase II amplitude of I amp (Estim). Note, the amplitude and phasic timing of the mathematically isolated I amp (Estim, AP DA ) was equal to that of the total I amp (Estim) in the presence of 10 μM MEC. ( d ) Summary of the I amp (Lstim) and I amp (Estim) with and without 10 μM MEC, as well as I amp (Estim, AP DA ). The data shown in panels b – d were from the same cells ( n =11). *** P <0.001, paired t -test. Data are mean±s.e.m. Full size image Next, we isolated the phase I component I amp (Estim, AP DA ) from I amp (Estim) (‘AP DA ’ denotes AP of dopaminergic axons). The same source and phasic timing of I amp (Lstim) and I amp (Estim, ChI) enabled us to estimate the I amp (Estim, ChI) by I ′ amp (Lstim), which was normalized I amp (Lstim) according to the amplitude of the phase II component of I amp (Estim). This resulted in the pure phase I component I amp (Estim, AP DA ) ( I amp (Estim, AP DA )= I amp (Estim)− I ′ amp (Lstim), Fig. 3c ). The result that I amp (Estim, AP DA ) was equal to the total I amp (Estim) in the presence of MEC ( Fig. 3c,d ) confirmed the reliability of the isolation. Nicotine bypasses DAergic AP-dependent DA release We next investigated the effect of physiologically relevant levels of nicotine on local Estim-induced DA release from both pathways. After pretreatment with 200 nM nicotine for ≤10 min in the slice, the Estim-induced DA release I amp was inhibited by 35±5% ( Fig. 4a left), while Lstim-induced DA release was fully blocked ( Figs 1c and 4a right). Remarkably, like the effect of the nAChR antagonist MEC shown in Fig. 3b , nicotine exposure selectively blocked the phase II component but not the phase I component of I amp (Estim) ( Fig. 4a , left), suggesting that only the Estim-induced DA release via the ChI pathway was blocked by the physiologically relevant levels of nicotine. Further, we determined whether physiologically relevant levels of nicotine had any effect on the dopaminergic AP-dependent DA release. We isolated the phase I component I amp (Estim, AP DA ) (dopaminergic AP-dependent DA release) from the total I amp (Estim) with and without nicotine (as described in Fig. 3c ). I amp (Estim, AP DA ) was 69±5% of control I amp (Estim) before pretreatment with nicotine, and 64±5% of control I amp (Estim) after the pretreatment, indicating that 200 nM nicotine had no effect on I amp (Estim, AP DA ), and that the Estim-induced DA release after nicotine pretreatment was entirely driven by AP firing of dopaminergic axons but not ChIs ( Fig. 4b,c ). Thus, Estim-induced DA release I amp (Estim) included both a phase I component I amp (Estim, AP DA ) representing for dopaminergic AP-dependent DA release and a phase II component I amp (Estim, ChI) representing for ChI-driven DA release. Physiologically relevant levels of nicotine selectively blocked the ChI-driven DA release, probably by desensitizing the nAChRs on the dopaminergic terminals, but nicotine did not affect the DA release evoked by given APs of dopaminergic axons ( Fig. 4d ). 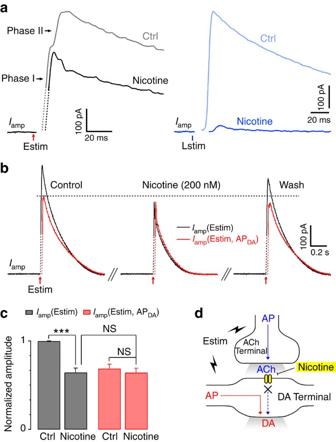Figure 4: Physiologically relevant levels of nicotine do not affect dopaminergic AP-dependent DA release. (a) After pretreatment with nicotine (200 nM) for 5–10 min, phase II ofIamp(Estim) was blocked, while the phase I component remained intact asIamp(Estim, APDA)=Iamp(Estim, nicotine) (left). For clarity, a horizontal offset was added to the black trace. In the same experiment, Lstim-induced ChI-driven DA release was abolished by nicotine (200 nM; right). (b) Nicotine (200 nM) reversibly and partially blocked the total DA release signalIamp(Estim), but not its phase I signalIamp(Estim, APDA). For clarity, a short horizontal offset was added toIamp(Estim, APDA). (c) Summary of the effect of nicotine onIamp(Estim) andIamp(Estim, APDA). The data shown in panelsa–cwere from the same cells (n=9). (d) Cartoon showing how nicotine affects Estim-induced DA release. Estim activates both the dopaminergic axons and the somata/axons of ChIs. Nicotine selectively blocks DA release from the ChI pathway by desensitizing α6β2* nAChRs on the dopaminergic terminals, while DA release driven by AP firing of dopaminergic axons remains intact. ***P<0.001, pairedt-test. Data are mean±s.e.m. Figure 4: Physiologically relevant levels of nicotine do not affect dopaminergic AP-dependent DA release. ( a ) After pretreatment with nicotine (200 nM) for 5–10 min, phase II of I amp (Estim) was blocked, while the phase I component remained intact as I amp (Estim, AP DA )= I amp (Estim, nicotine) (left). For clarity, a horizontal offset was added to the black trace. In the same experiment, Lstim-induced ChI-driven DA release was abolished by nicotine (200 nM; right). ( b ) Nicotine (200 nM) reversibly and partially blocked the total DA release signal I amp (Estim), but not its phase I signal I amp (Estim, AP DA ). For clarity, a short horizontal offset was added to I amp (Estim, AP DA ). ( c ) Summary of the effect of nicotine on I amp (Estim) and I amp (Estim, AP DA ). The data shown in panels a – c were from the same cells ( n =9). ( d ) Cartoon showing how nicotine affects Estim-induced DA release. Estim activates both the dopaminergic axons and the somata/axons of ChIs. Nicotine selectively blocks DA release from the ChI pathway by desensitizing α6β2* nAChRs on the dopaminergic terminals, while DA release driven by AP firing of dopaminergic axons remains intact. *** P <0.001, paired t -test. Data are mean±s.e.m. Full size image Nicotine reduces depletion of DA vesicle pool To test whether nicotine affects depletion of the DA vesicle pool (termed ‘DA depletion’), we did the paired-pulse ratio test [27] , [28] and estimated the DA depletion level after paired pulses of Lstim–Estim at intervals from 0.05 to 120 s. I amp (Estim, AP DA ) at 1 s interval after the preceding Lstim was suppressed by 75±2% of I amp (Estim 0 , AP DA ). I amp (Estim 0 , AP DA ) was the phase I of DA release evoked by Estim when vesicle pool was full ( Fig. 5a ). The depletion level was increased when the interval was reduced within 60 s. The maximum depletion of 82±3% was obtained at the shortest tested interval of 0.05 s ( Fig. 5c ). These results suggested that at least 80% of the DA vesicle pool in the dopaminergic AP-dependent DA release was depleted by the preceding cholinergic transmission. The depletion level was estimated by ( I amp (Estim 0 , AP DA )− I amp (Estim, AP DA ))/ I amp (Estim 0 , AP DA ) × 100%. After pretreatment with nicotine, the DA depletion level at the 0.5-s interval after Lstim was dramatically reduced from 76±2% (control) to 3.7±5% (nicotine) ( Fig. 5b,d ). These data suggested that the DA depletion of dopaminergic AP-dependent release following cholinergic transmission was eliminated by physiologically relevant levels of nicotine. 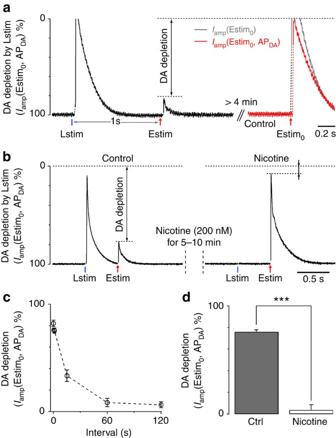Figure 5: Physiologically relevant levels of nicotine reduce depletion of DA vesicle pool by blocking ChI-driven DA release. (a) Paired pulses of Lstim–Estim revealed that cholinergic excitation induced a large percentage of DA vesicle pool depletion (≥75±2%, defined by ΔIamp(Estim, APDA)/Iamp(Estim0, APDA) × 100% ) of the DA vesicle pool for dopaminergic AP-dependent DA release. The phase I componentIamp(Estim, APDA) in the totalIamp(Estim) was predicted by component isolation for intervals >1 s (seeFig. 3c). The Estim at rest (>4 min before or after the paired stimulation) was used as the control pulse (Estim0).Iamp(Estim, APDA) was equal toIamp(Estim) at the intervals 0.05–1 s (data not shown). For clarity, a short horizontal offset was added to controlIamp(Estim0, APDA). (b) In this experiment, the paired Lstim–Estim protocol (1 s interval) was tested before or after 200 nM nicotine treatment. Before nicotine application, Lstim induced a large DA release and caused DA vesicle pool depletion (76±2%=Iamp(Estim0, APDA)−Iamp(Estim, APDA)/Iamp(Estim0, APDA)). After nicotine application (200 nM, pretreatment for 5–10 min), Lstim caused neither DA release (Iamp(Lstim)=0) nor DA vesicle pool depletion. (c) DA depletion ofIamp(Estim, APDA) was correlated with the interval between Lstim and Estim (n=7 to 8 at different intervals). (d) The DA depletion ofIamp(Estim, APDA) was 76±2% in the control versus 3.7±5% with nicotine (n=6). ***P<0.001, pairedt-test. Data are mean±s.e.m. Figure 5: Physiologically relevant levels of nicotine reduce depletion of DA vesicle pool by blocking ChI-driven DA release. ( a ) Paired pulses of Lstim–Estim revealed that cholinergic excitation induced a large percentage of DA vesicle pool depletion (≥75±2%, defined by Δ I amp (Estim, AP DA )/ I amp (Estim 0 , AP DA ) × 100% ) of the DA vesicle pool for dopaminergic AP-dependent DA release. The phase I component I amp (Estim, AP DA ) in the total I amp (Estim) was predicted by component isolation for intervals >1 s (see Fig. 3c ). The Estim at rest (>4 min before or after the paired stimulation) was used as the control pulse (Estim 0 ). I amp (Estim, AP DA ) was equal to I amp (Estim) at the intervals 0.05–1 s (data not shown). For clarity, a short horizontal offset was added to control I amp (Estim 0 , AP DA ). ( b ) In this experiment, the paired Lstim–Estim protocol (1 s interval) was tested before or after 200 nM nicotine treatment. Before nicotine application, Lstim induced a large DA release and caused DA vesicle pool depletion (76±2%= I amp (Estim 0 , AP DA )−I amp (Estim, AP DA )/ I amp (Estim 0 , AP DA )). After nicotine application (200 nM, pretreatment for 5–10 min), Lstim caused neither DA release ( I amp (Lstim)=0) nor DA vesicle pool depletion. ( c ) DA depletion of I amp (Estim, AP DA ) was correlated with the interval between Lstim and Estim ( n =7 to 8 at different intervals). ( d ) The DA depletion of I amp (Estim, AP DA ) was 76±2% in the control versus 3.7±5% with nicotine ( n =6). *** P <0.001, paired t -test. Data are mean±s.e.m. Full size image Facilitation of phasic DA release by nicotine Finally, we investigated the effect of physiologically relevant levels of nicotine on bursts of Estim-induced DA release using a train of 10 pulses at 20 Hz. In contrast to the inhibitory effect of nicotine on the DA release induced by a single pulse of Estim which simultaneously activated both the ascending dopaminergic axons and striatal ChIs ( Fig. 4 ), the DA release induced by the second and the third pulses during a burst of Estim showed facilitation in the presence of nicotine ( Fig. 6a ). For quantitative analysis, we used the forward-interpolation method to calculate the amplitude of the evoked DA release and defined the ‘total DA release’ as the sum of the individual I amp (Estim) peaks, ( N is the pulse number, N =1 or 10). Like the data shown in Fig. 4 , nicotine inhibited the DA release induced by single pulse of Estim ( N =1) by 35±5%; however, the nicotine-induced inhibition of DA release was significantly attenuated to 16±7% when the total DA release was induced by a burst of Estim ( N =10; Fig. 6d ). The contrast of phasic DA release versus tonic DA release is represented by the proportion of a burst of Estim-induced DA release to single Estim-induced DA release (that is, ). The contrast was increased from 1.88±0.28 (control) to 2.47±0.41 (nicotine; Fig. 6e ). Note that the nicotine enhancement of the phasic-versus-tonic contrast of DA release depended on the high frequency of Estim to keep the DA vesicle pool in high depletion level at each pulse. When the stimulation frequency was low (<0.1 Hz), the later pulses triggered the same DA release as the preceding pulse, and the nicotine enhanced contrast disappeared (data not shown). Thus, the effect of nicotine on burst DA release depended on stimulation frequency, which is consistent with previous studies [7] , [8] . 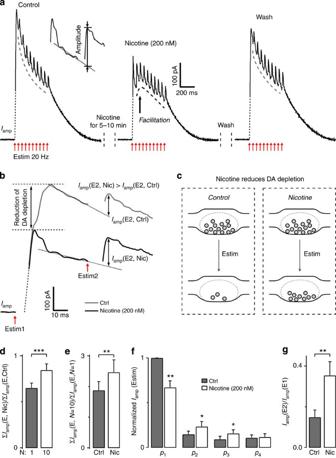Figure 6: Physiologically relevant levels of nicotine permit facilitation of sustained DA release following a burst of Estim. (a) In the typical striatal slice recording, nicotine (200 nM) permitted the facilitation of DA release induced by a 20-Hz burst of Estim. Inset: evoked change inIampamplitude measured by forward-interpolation of the decaying baseline. Note: in addition to its facilitatory effect on the within-burst DA release, nicotine reversibly inhibited the interburst DA release induced by the first Estim pulse (E1),Iamp(E1, Nic)<Iamp(E1, Ctrl). (b) Physiologically relevant levels of nicotine (200 nM) blocked phase II component of Iamp(E1, Ctrl), while it enhanced the second release peak,Iamp(E2, Nic)>Iamp(E2, Ctrl). (c) Cartoon showing how physiologically relevant levels of nicotine reduces DA vesicle depletion. (d) Summary of nicotinic modulation of DA release induced by a 20-Hz burst of Estim versus a single pulse of Estim.(N=1 or 10) is the sum of the amplitude of allIamp(Estim) at each pulse during a burst.Nis the total number of pulses. Nicotinic inhibition was 16±7% for a burst of Estim (N=10 at 20 Hz), while it was 35±5% for a single Estim (N=1). (e) Summary of the nicotine-enhanced contrast of DA release between burst Estim (N=10 at 20 Hz) and a single Estim (N=1). (f) The effect of nicotine on the first four peaks (p1–p4) of Estim-induced burst DA release (normalized toIamp(E1, Ctrl)). (g) Summary of the effect of nicotine on the paired-pulse ratio (PPR=Iamp(E2)/Iamp(E1)) of the DA release induced by the first two Estim pulses in panelb. The data shown in all panels were from the same cells (n=7, pairedt-test). *P<0.05, **P<0.01, ***P<0.001, pairedt-test. Data are mean±s.e.m. Figure 6: Physiologically relevant levels of nicotine permit facilitation of sustained DA release following a burst of Estim. ( a ) In the typical striatal slice recording, nicotine (200 nM) permitted the facilitation of DA release induced by a 20-Hz burst of Estim. Inset: evoked change in I amp amplitude measured by forward-interpolation of the decaying baseline. Note: in addition to its facilitatory effect on the within-burst DA release, nicotine reversibly inhibited the interburst DA release induced by the first Estim pulse (E1), I amp (E1, Nic)< I amp (E1, Ctrl). ( b ) Physiologically relevant levels of nicotine (200 nM) blocked phase II component of I amp (E1, Ctrl), while it enhanced the second release peak, I amp (E2, Nic)> I amp (E2, Ctrl). ( c ) Cartoon showing how physiologically relevant levels of nicotine reduces DA vesicle depletion. ( d ) Summary of nicotinic modulation of DA release induced by a 20-Hz burst of Estim versus a single pulse of Estim. ( N =1 or 10) is the sum of the amplitude of all I amp (Estim) at each pulse during a burst. N is the total number of pulses. Nicotinic inhibition was 16±7% for a burst of Estim ( N =10 at 20 Hz), while it was 35±5% for a single Estim ( N =1). ( e ) Summary of the nicotine-enhanced contrast of DA release between burst Estim ( N =10 at 20 Hz) and a single Estim ( N =1). ( f ) The effect of nicotine on the first four peaks ( p 1 – p 4 ) of Estim-induced burst DA release (normalized to I amp (E1, Ctrl)). ( g ) Summary of the effect of nicotine on the paired-pulse ratio (PPR= I amp (E2)/ I amp (E1)) of the DA release induced by the first two Estim pulses in panel b . The data shown in all panels were from the same cells ( n =7, paired t -test). * P <0.05, ** P <0.01, *** P <0.001, paired t -test. Data are mean±s.e.m. Full size image We further assessed the effect of nicotine on each peak of the DA release induced by a burst of Estim. In the presence of physiologically relevant levels of nicotine, evoked DA release during a burst of stimulation was inhibited at the first pulse I amp (E1, Nic)< I amp (E1, Ctrl), but then was facilitated at the second pulse I amp (E2, Nic)> I amp (E2, Ctrl) ( Fig. 6b,f ). However, only the phase II component of the first peak was inhibited, but the phase I component of the first peak was intact, suggesting that the ChI-driven DA release but not the dopaminergic AP-dependent DA release was blocked by nicotine, meanwhile the depletion of the DA vesicle pool was reduced ( Fig. 6b,c ). Surprisingly, but consistent with observations by others [7] , [8] , the DA release evoked by the second and the third pulses was facilitated ( Fig. 6b,f ), and the paired-pulse ratio of the release induced by the first two pulses rose from 0.15±0.03 (control) to 0.35±0.07 (nicotine; Fig. 6g ). Thus, by selectively suppressing DA release via the ChI pathway, and reducing the depletion of the DA vesicle pool, physiologically relevant levels of nicotine caused the facilitation of phasic DA release. These results revealed the mechanism underlying the paradoxical observations of single pulse inhibition and burst-pulses facilitation of DA release in the striatum by physiologically relevant levels of nicotine. We demonstrated that local Estim triggered not only the dopaminergic AP-dependent DA release but also the ChI-driven DA release. With selective optogenetic stimulation on ChIs in the dorsal striatum, we found that physiologically relevant levels of nicotine potently inhibited the ChI-driven DA release. Nicotine did not affect the DA release driven by given APs of dopaminergic axons, but reduced the ChI-induced depletion of the DA vesicle pool, and therefore permitted the facilitation of sustained DA release during a burst of Estim. The major discovery of the present work is that physiologically relevant levels of nicotine modulates DA release by selectively blocking the DA release driven by AP of ChIs but not the release driven by AP of dopaminergic axons. This is based on the following evidence: (1) single Estim-induced DA release contained phase I and phase II components ( Fig. 3a ); (2) the phase I component I amp (Estim, AP DA ) reflected the MEC-insensitive dopaminergic AP-dependent DA release and the phase II component I amp (Estim, ChI) reflected the MEC-sensitive ChI-driven DA release ( Fig. 3b ); (3) Lstim-induced ChI-driven DA release was suppressed by physiologically relevant levels of nicotine ( Fig. 1c,d,f ); (4) Lstim-induced ChI-driven DA release was suppressed by ambenonium, which inhibits acetylcholinesterase and causes the accumulation of extracellular ACh ( Fig. 1e ); and (5) physiologically relevant levels of nicotine inhibited the phase II component but not the phase I component of DA release induced by Estim ( Fig. 4 ). Note, in addition to dopaminergic and cholinergic transmissions, local Estim could co-activate other types of synaptic transmission such as GABAergic and glutamatergic transmissions, but previous works do not show significant effect of GABAergic and glutamatergic transmission on regulating DA release in the dorsal striatum [7] , [8] , [29] . The long-held view of nicotinic modulation of the DA signal is based on the DA release evoked by Estim, which assumes that DA release is exclusively induced by stimulating the dopaminergic axons [6] , [7] , [8] , [17] . We found that physiologically relevant levels of nicotine selectively inhibited the ChI-driven DA release, but had no significant effect on the dopaminergic AP-dependent DA release ( Fig. 4 ). We revealed that the major nAChRs mediating ChI-driven DA release included α6 and β2 subunits ( Fig. 2 ). Although both α3 and α6 subunits are sensitive to α-ctx MII, the α3-subunit is poorly expressed in the striatum [18] , [20] . α-ctx MII also has a negligible effect on α4(non-α6)β2* nAChRs [18] , [20] . Thus, the inhibitory effect of α-ctx MII suggested that the α6 subunit was involved in 87±3% of the nAChRs-mediated DA release. In addition, blocking ionotropic glutamate receptors with CNQX and D-APV or muscarinic ACh receptors with atropine had little effect on Lstim-induced DA release (data not shown). Thus, α6* nAChRs play the predominant postsynaptic role in mediating ChI-driven DA release in the dorsal striatum ( Fig. 2a ). nAChRs have been considered to regulate striatal DA release and modulate locomotor activity, as well being involved in nicotine self-administration [6] , [8] , [17] , [23] , [30] . However, the contribution of α6* nAChRs to the modulation of DA release in the dorsal striatum is controversial. Lester’s group reported that α6* nAChRs have an important function to regulate DA transmission and locomotor activity [17] , [23] , while Cragg’s group reported that α4α5(non-α6)β2* nAChRs predominantly regulate DA transmission [24] . In the present work, we determined that α6β2* nAChRs mediated 87% of DA release via the ChI pathway ( Fig. 2 ). Synaptic facilitation requires two preconditions: (1) terminal [Ca 2+ ] i accumulation during a burst of stimulation; and (2) sufficient releasable vesicles remaining in the presynaptic terminals after the first of paired stimuli [13] , [31] , [32] . Actually, facilitation is usually masked by depression and becomes evident only when the depression is relieved by reducing the amount of vesicular transmitter release [33] . In the absence of nicotine, precondition (1) was achieved during high-frequency stimulation, while the precondition (2) was not. The first pulse of a burst of stimuli induced a high percentage of vesicular DA release and the vesicle pool was subsequently depleted, which caused short-term depression ( Fig. 6a ). In the presence of nicotine, the vesicle pool was less depleted ( Fig. 5b ), which permitted the facilitation of DA release when Ca 2+ accumulated during a burst of Estim ( Fig. 6a,b , see also refs 7 , 8 ). Thus, physiologically relevant levels of nicotine permit the frequency-dependent facilitation of DA release. In a previous study, Dani’s group found that nicotine inhibits DA release following tonic Estim [6] , while Sulzer’s and Cragg’s groups reported that nicotine enhances phasic DA release and the contrast between the phasic and the tonic release and thus provide an interpretation for nicotinic facilitation of reward-related DA signals [7] , [8] . These apparently paradoxical observations on nicotinic modulation of Estim-induced DA release can now be interpreted on the basis of our findings: (1) local Estim stimulated both dopaminergic axons and striatal ChIs in striatal slices ( Fig. 3 ); (2) physiologically relevant levels of nicotine selectively blocked the ChI pathway by desensitizing α6β2* nAChRs on the dopaminergic terminals, which caused the inhibition of DA release following a single pulse of Estim (mimicking low-frequency tonic firing; Figs 1 and 4 ); and (3) physiologically relevant levels of nicotine caused short-term facilitation of DA release at the second and the third pulses in the 20-Hz burst of Estim (mimicking high-frequency phasic firing) because blockade of the ChI pathway reduced the depletion of the DA vesicle pool at the first pulse in a train of Estim ( Figs 5 and 6 ). DA system is profoundly involved in psychostimulant drug addiction such as nicotine administration in cigarette smoking. Blocking DA transmission in the ventral striatum reduces the nicotine self-administration, suggesting that DA plays an essential role in rewarding [34] . In addition to its modulation on APs of dopaminergic somata [2] , [35] , [36] , nicotine is also thought to directly regulate the downstream DA release [6] , [7] , [8] , [17] . However, this current view does not consider the role of ChIs in directly triggering DA release in both ventral and dorsal striatum [17] . In the present work, we demonstrated that the widely used local Estim in striatal slices evokes DA release by stimulating not only dopaminergic axons, but also ChIs ( Fig. 3 ). The ChI-driven DA release was extremely sensitive to acute physiologically relevant levels of nicotine ( Fig. 1c,d,f ). Although DA release by given APs of dopaminergic axons was not affected by acute nicotine exposure ( Fig. 4 ), the APs of midbrain dopaminergic neurons can be modulated by nicotine [2] , [17] , [35] , [36] . Thus, the current view about nicotine modulation of DA release needs to add the ChI-driven pathway. In summary, we show that nicotine abolishes the ChI-driven DA release but not the dopaminergic AP-dependent DA release in the dorsal striatum. Through reduction of the depletion of DA vesicle pool, nicotine also facilitated the burst DA release. Thus, physiologically relevant levels of nicotine modulate striatal DA release through α6β2* nAChRs of the ChI pathway. Animals All experimental mice were used according to protocols approved by the Peking University Institutional Animal Care and Use Committee (Approval ID: IMM-zhouz-11). All experiments were performed on ChAT-ChR2-EYFP transgenic mice (line 6, 3–12 weeks old) of either sex. In these mice, the expression of ChR2(H134R)-EYFP (termed ChR2-EYFP) is driven by the promoter of choline acetyltransferase (ChAT) [37] , [38] . For patch-clamp recordings, we used mice 3–4 weeks old. Immunohistochemistry Immunofluorescence was performed as previously described [39] . Briefly, adult mice were anesthetized as described [40] and prefixed with 4% paraformaldehyde through transcardial perfusion. The brain was removed, postfixed in 4% paraformaldehyde overnight at 4 °C and then equilibrated in 30% sucrose. Horizontal sections were cut at 50 μm on a cryostat. Free-floating sections were washed in PBS and incubated for 1 h at room temperature in 2% bovine serum albumin in PBS containing 0.2% Triton X-100. Sections were then incubated for 24 h at 4 °C with primary antibody in bovine serum albumin. The primary antibodies were goat anti-ChAT (1:500, Millipore), rabbit anti-VAChT (1:500, Synaptic Systems) and rabbit anti-TH (1:500, Millipore). After being washed in PBS, sections were incubated with a secondary antibody for 3 h in the dark at room temperature. The secondary antibodies were Alexa546-conjugated donkey anti-goat (1:500, Life Technologies) and Alexa594-conjugated goat anti-rabbit (1:333, Life Technologies). Sections were then washed, stained with 1 μM 4',6-diamidino-2-phenylindole (Life Technologies), and mounted on slides with mounting solution (Dako). Fluorescent images were acquired on an upright confocal laser-scanning microscope (Zeiss LSM 700, Carl Zeiss) with a × 40 water-immersion objective. Slice preparation and electrophysiological recording Horizontal slices through the striatum were prepared as described previously [37] , [39] , [41] with minor modifications. Mice were anesthetized as described [40] and transcardially perfused with 5–10 ml ice-cold cutting solution containing (in mM): 92 N -methyl- D -glucamine, 2.5 KCl, 0.5 CaCl 2 , 10 MgSO 4 , 1.2 NaH 2 PO 4 , 30 NaHCO 3 , 25 glucose, 20 HEPES, 5 ( L )-ascorbic acid and 3 Na-pyruvate (adjusted to pH 7.3–7.4 with concentrated HCl, saturated with 95% O 2 and 5% CO 2 ). Horizontal slices (300 μm thick) were cut on a vibratome (VT1200s, Leica), allowed to recover for 10–15 min at 33 °C in cutting solution, then incubated for at least 1 h at room temperature in artificial cerebrospinal fluid (ACSF) before electrophysiological recording. The ACSF contained (in mM): 112 NaCl, 2.5 KCl, 2 CaCl 2 , 2 MgSO 4 , 1.2 NaH 2 PO 4 , 30 NaHCO 3 , 12.5 glucose and 20 HEPES (saturated with 95% O 2 and 5% CO 2 ). Supplements of 5 mM ( L )-ascorbic acid, 3 mM Na-pyruvate, 100 units ml −1 penicillin G sodium and 100 μg ml −1 streptomycin sulphate were added to the ACSF for incubation. Slices were superfused (1–2 ml min −1 ) with ACSF (without the supplements) during the subsequent electrophysiological experiments. Cells were visualized under an upright microscope (BX51WI, Olympus) equipped with infrared and differential interference contrast imaging devices, and with a × 60 water-immersion objective. We used an EPC9/2 amplifier (HEKA Elektronik) to obtain whole-cell patch-clamp recordings as described previously [39] , [42] . The resistances of the patch electrodes were 3–4 MΩ when filled with internal solution that contained (in mM): 130 K-gluconate, 5 KCl, 4 MgCl 2 , 10 HEPES, 10 Na 2 -phosphocreatine, 0.2 EGTA, 2 Mg-ATP and 0.4 Na 3 -GTP (adjusted to pH 7.2 with KOH). Signals were digitalized at 20 kHz and low-pass filtered at 2.9 kHz. Amperometric recordings Amperometric recordings in dorsal striatum slices were performed as previously described [12] , [13] , [39] . CFEs (Dagan Instruments, Minneapolis, USA) 7 μm in diameter were used to measure DA release. The length of the exposed tip inserted into the subsurface of the striatal slice was 200–300 μm. A holding potential of 780 mV was applied to the electrode by an EPC9/2 amplifier. The amperometric current ( I amp ) was low-pass filtered at 100 Hz and digitized at 3.13 kHz. Optogenetic and electrical stimulation We used a 470-nm light-emitting diode (Yibo Instruments Inc., China) for optogenetic Lstim following the standard procedure [43] . The output of the light-emitting diode was coupled to the microscope and focused onto a spot of the tissue (440 μm in diameter) by a × 60 water-immersion objective. The maximal light intensity reaching the tissue was ~\n4.2 mW mm −2 . Because of the universal and relative even expression of ChR2 throughout the dorsal striatum, we usually perform high successful rate blind recordings without visualizing the fluorescence of EYFP in ChAT-ChR2-EYFP positive mice. When visualizing the fluorescence of EYFP of ChIs in brain slices, we used the 488 nm visible light from a monochromator (T.I.L.L. Photonics) with a 15%-reflection beam-splitter. Bipolar platinum electrodes (150 μm in diameter) with a tip separation of 20 μm were used for Estim. The bipolar electrodes were placed on the surface of the slice, parallel to the CFE and 100 μm from the sensor tip of the CFE. Single pulses (0.2 ms, 0.3–1.4 mA) generated by a stimulator with an isolation unit (S88K, Grass Instruments) were used to evoke DA release. Both Lstim and Estim were triggered by 5-V TTL signals from the EPC9/2 amplifier. Drugs and data analysis Dihydro-β-erythroidine hydrobromide, α-ctx MII and ambenonium were from Tocris Bioscience. All other drugs used in this study were from Sigma-Aldrich except where specifically noted. A drug-puffing device (MPS1, Yibo Instruments Inc., Wuhan, China) was used to deliver drugs to the recording site under study. IGOR Pro 6.22 software (Wavemetrics) was used for data analysis. Stimulation-induced transient artifacts in amperometric traces were removed for clarity. Data are presented as mean±s.e.m. Statistical significance was determined by Student’s t -test. A difference was considered significant at P <0.05. How to cite this article: Wang, L. et al. Modulation of dopamine release in the striatum by physiologically relevant levels of nicotine. Nat. Commun. 5:3925 doi: 10.1038/ncomms4925 (2014).